Lymph node-independent liver metastasis in a model of metastatic colorectal cancer Deciphering metastatic routes is critically important as metastasis is a primary cause of cancer mortality. In colorectal cancer (CRC), it is unknown whether liver metastases derive from cancer cells that first colonize intestinal lymph nodes, or whether such metastases can form without prior lymph node involvement. A lack of relevant metastatic CRC models has precluded investigations into metastatic routes. Here we describe a metastatic CRC mouse model and show that liver metastases can manifest without a lymph node metastatic intermediary. Colorectal tumours transplanted onto the colonic mucosa invade and metastasize to specific target organs including the intestinal lymph nodes, liver and lungs. Importantly, this metastatic pattern differs from that observed following caecum implantation, which invariably involves peritoneal carcinomatosis. Anti-angiogenesis inhibits liver metastasis, yet anti-lymphangiogenesis does not impact liver metastasis despite abrogating lymph node metastasis. Our data demonstrate direct hematogenous spread as a dissemination route that contributes to CRC liver malignancy. Colorectal cancer (CRC) initially manifests as benign adenomatous polyps on the mucosal surface of the large intestine. If left unresected, these polyps can progress to invasive adenocarcinomas, that penetrate through the submucosal and muscularis externa layers of the colorectal wall to reach the serosal side. Eventual regional spread to the intestinal lymph nodes and distant spread to the liver results in the outgrowth of gross metastases that are the major cause of CRC mortality. It is currently unknown whether distant CRC metastases in the liver derive from cancer cells that have first colonized the regional intestinal lymph nodes after accessing the lymphatic vasculature, or whether these liver metastases can form without prior outgrowth in regional lymph nodes [1] . Deciphering the routes of CRC metastasis to these sites has the potential to uncover therapeutic opportunities that may impact CRC mortality rates. Investigations into CRC metastatic routes, however, have been precluded by the lack of availability of relevant in vivo metastatic models of CRC. Indeed, despite the wide availability of xenograft, chemical-induced and genetically-engineered mouse models of CRC [2] , [3] , [4] , [5] , tumours in these models fail to reproducibly metastasize to the regional intestinal lymph nodes and liver—the target organs relevant to human CRC. The most widely utilized genetically-engineered mouse model of intestinal cancer is the Apc Min/+ mouse, which harbours a dominant nonsense mutation in one Apc allele [6] . Apc Min/+ mice develop numerous adenomas within the intestinal tract; however, these adenomas rarely, if ever, progress to invasive or metastatic adenocarcinomas [7] . Moreover, these adenomas primarily localize to the small intestine, with relatively few adenomas manifesting in the colon [7] . Introduction of oncogenic Kras to the mutant Apc background promotes intestinal adenoma multiplicity [8] , [9] and accelerates progression to invasiveness [8] , [10] , [11] , with a marked enhancement of tumour development in the relevant anatomical location of the colon [9] . Development of intestinal lymph node metastases, however, has not been observed in Apc/Kras compound mutant mice [8] , [12] , with distant liver metastases only detected in 20–27% of Apc/Kras compound mutant mice by transgene RT–PCR [8] or gross observation [12] . Of note, Apc/Kras compound mutant mice exhibit a dramatically reduced lifespan, which can be attributed to intestinal tumour overburden [9] , [10] . Given that Apc/Kras compound mutant tumours exhibit features of early-stage malignant progression [8] , [10] , [11] , we postulated that maintaining a compound mutant tumour in vivo beyond the shortened lifespan of an Apc/Kras mutant mouse might enable a realization of metastatic potential. We therefore sought to transplant a single intact Apc/Kras compound mutant donor tumour within the mucosal layer of a host wild-type C57BL/6J mouse colon, as this would faithfully represent an orthotopic primary colorectal tumour at clinical stage 0 (in situ carcinoma) with the potential to progress to stage IV disease. Several colon orthotopic transplantation techniques have been described to date, including the injection of cancer cell suspensions directly into the rectal mucosa [13] or serosal wall of the caecum [14] , the instillation of tumour cell suspensions into the colonic lumen following electrocoagulation of the mucosa to promote tumour cell uptake [15] , and the surgical implantation of intact tumour fragments onto the serosal side of the caecal wall [16] , [17] . One drawback of caecum implantation is the fact that tumours are implanted on the serosal side of the caecal wall, thus bypassing the requirement of primary tumour invasion through the mucosa to the serosa for metastasis to occur. Importantly, a major caveat of all of these established techniques is the potential for inadvertent seeding of tumour cells into the peritoneal space, whether from a breach of the colon wall during tumour cell injection into the mucosa, or from the shedding of tumour cells from the caecal implant following return to the peritoneal cavity. Indeed, although these techniques have been utilized to generate mouse models of CRC that reportedly develop metastases in the intestinal lymph nodes, liver and lungs, these techniques also give rise to widespread peritoneal carcinomatosis [14] , [15] , [16] , [17] . It is thus highly plausible that tumour formation in these secondary sites may not be true metastases, but rather a result of peritoneal seeding. The fact that peritoneal carcinomatosis is not a prominent feature of human metastatic CRC [18] further suggests a limited utility of these models for investigating routes of metastatic dissemination. Here we describe a mouse model of metastatic CRC that exhibits tumour cell dissemination to specific target organs, including the intestinal lymph nodes, liver and lungs. Using this model to directly interrogate routes of metastatic spread, we demonstrate that CRC liver metastases can manifest in the absence of an intestinal lymph node metastatic intermediary. Benign colon tumours from Apc/Kras compound mutant mice Given that colorectal tumours from Apc/Kras compound mutant mice develop features of early-stage malignant progression [8] , [10] , [11] , we sought to utilize these tumours in an attempt to develop a reproducible model of metastatic CRC for investigating routes of metastatic dissemination. We generated Apc Min/+ ;Kras LSLG12D/+ ;Villin-Cre compound mutant mice (mice carrying a Cre-dependent activated allele of Kras ( Kras LSLG12D ) on the Apc Min/+ background, crossed with mice carrying a Villin-Cre transgene that directs expression of Cre recombinase throughout the intestine), and confirmed an enhancement of tumour development in the colon compared with Apc Min/+ ;Villin-Cre control mice ( Supplementary Fig. 1a–c ). As a consequence of accelerated intestinal tumorigenesis, however, Apc Min/+ ;Kras LSLG12D/+ ;Villin-Cre mice exhibited a dramatically reduced lifespan ( Supplementary Fig. 1d ), consistent with previous reports [9] , [10] . As expected, disease status at the onset of morbidity at ~9 weeks of age remained benign, as evidenced by primary colon tumours that failed to invade through to the serosal side of the colon wall and a lack of metastasis formation in the liver ( Supplementary Fig. 1b ). We next sought to develop a technique that would allow us to maintain a compound mutant tumour in vivo beyond the shortened lifespan of an Apc/Kras mutant mouse, as this might enable a realization of metastatic potential. To this end, we developed a rectal prolapse induction technique that exteriorizes the lumen of the host colon, thus rendering the colonic mucosal surface amenable to surgical manipulation ( Fig. 1a ). Using donor tumours from 6–9-week-old Apc Min/+ ;Kras LSLG12D/+ ;Villin-Cre mice or wild-type C57BL/6J mice bearing subcutaneous Apc Min/+ ;Kras LSLG12D/+ ;Villin-Cre allograft tumours, we surgically implanted single intact donor colon tumours into wild-type C57BL/6J host colons. Of note, donor tumours were not dissociated to single cells before implantation, but rather were maintained as intact tumour tissues as this would preserve interactions of tumour cells with both stromal cells and extracellular matrix components. These intact donor tumours became established within the mucosal layer and exhibited long-term persistence in vivo as evidenced by serial endoscopy ( Supplementary Fig. 1e ) or gross imaging ( Supplementary Fig. 1f ). At host mouse death due to age-related morbidity, the vast majority of implanted donor tumours remained benign ( Fig. 1b and Supplementary Fig. 1e,f ), while only 3 of 17 (17.6%) mice exhibited malignant progression with donor tumour invasion through the colon wall and concommitant intestinal lymph node and liver metastasis formation at 51–92 weeks post implantation (w.p.i. ; Fig. 1c and Supplementary Fig. 1g ). These findings highlight the impractical use of benign adenomas for studying routes of metastatic spread, thus supporting a requirement for additional genetic, epigenetic and/or microenvironmental changes over a prolonged time period for tumour progression and metastasis to occur. 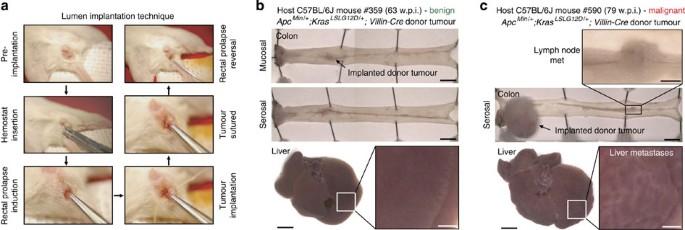Figure 1: Lumen-implanted endogenousApcMin/+;KrasLSLG12D/+;Villin-Crecolon tumours rarely progress to invasive and metastatic disease. (a) The lumen implantation technique. Details of the technique are provided in the Methods section. (b,c) Gross images of colons and livers from two host wild-type C57BL/6J mice that have received lumen implants of a single intactApcMin/+;KrasLSLG12D/+;Villin-Credonor tumour, harvested at 63 w.p.i. (b; host mouse #359; benign) or at 79 w.p.i. (c; host mouse #590; malignant). Colon mucosal and/or serosal views were imaged with the anus positioned to the left. Arrows indicate implanted donor tumours. Boxed areas of the liver have been enlarged. Boxed area of the colon inchas been enlarged to highlight a lymph node metastasis. Scale bars represent 5 mm (colon), 4 mm (liver), and 1 mm (liver boxed area and lymph node). Figure 1: Lumen-implanted endogenous Apc Min/+ ;Kras LSLG12D/+ ;Villin-Cre colon tumours rarely progress to invasive and metastatic disease. ( a ) The lumen implantation technique. Details of the technique are provided in the Methods section. ( b , c ) Gross images of colons and livers from two host wild-type C57BL/6J mice that have received lumen implants of a single intact Apc Min/+ ;Kras LSLG12D/+ ;Villin-Cre donor tumour, harvested at 63 w.p.i. ( b ; host mouse #359; benign) or at 79 w.p.i. ( c ; host mouse #590; malignant). Colon mucosal and/or serosal views were imaged with the anus positioned to the left. Arrows indicate implanted donor tumours. Boxed areas of the liver have been enlarged. Boxed area of the colon in c has been enlarged to highlight a lymph node metastasis. Scale bars represent 5 mm (colon), 4 mm (liver), and 1 mm (liver boxed area and lymph node). Full size image Invasion and metastasis of lumen-implanted colorectal tumours In an effort to shorten the timeframe of malignant progression in our model so that routes of metastasis could be interrogated, we applied our lumen implantation technique to the poorly-differentiated HCT116 human CRC-derived cell line. HCT116 cells were transduced with the gene encoding the red fluorescent protein DsRed, and implanted subcutaneously in a mouse to generate donor xenograft tumours. Following surgical implantation of donor tumour fragments of ~10 mm 3 onto the mucosal surface of host NOD/SCID mouse colons, ex vivo gross imaging ( Fig. 2a ) and in vivo endoscopy ( Fig. 2b ) were used to monitor tumour take rate and growth over time ( Fig. 2c ). Implanted tumours initially established and grew within the luminal space of the colon ( Fig. 2a,b ), with single tumour foci detectable as intramucosal carcinomas 1 w.p.i. ( Fig. 2d,e ). Histological assessment immediately post implantation confirmed that the implantation procedure did not breach the thickness of the colon wall, as primary tumours were localized exclusively on the mucosal surface of the colon ( Supplementary Fig. 2a,b,d,e ) with the integrity of the deeper wall layers maintained ( Supplementary Fig. 2c,f ). Flow cytometric analysis of the blood, liver, lungs and intestinal marginal vascular tract (encompassing the paracolic, intermediate and principal intestinal lymph nodes) one day post implantation confirmed the absence of disseminated HCT116-DsRed-positive cells at this early time point ( Supplementary Fig. 2g ). Stage 0 polyps invariably progressed to stage I tumours, which breached the submucosal/muscularis externa layers, such that by 2–3 w.p.i. invasive stage II adenocarcinomas that penetrated through the collagen IV-rich basement membrane of the muscularis externa to reach the serosal side of the colon wall were evident ( Fig. 2a and Supplementary Fig. 3 ). Of note, at 3 w.p.i., individual clusters of invasive tumour cells were detectable within the colon wall both adjacent to ( Fig. 2f–h ) and distant from ( Fig. 2f,i ) the primary adenocarcinoma. Continued expansion of the primary adenocarcinoma occurred predominantly on the serosal side of the colon wall ( Fig. 2a and Supplementary Fig. 3a ), to the extent that luminal obstruction was not evident even at the harvest endpoint of 7 w.p.i. Rather, animal morbidity at 7 w.p.i. was attributable primarily to weight loss due to primary tumour burden, a common symptom also observed in CRC patients with later stage disease [19] . 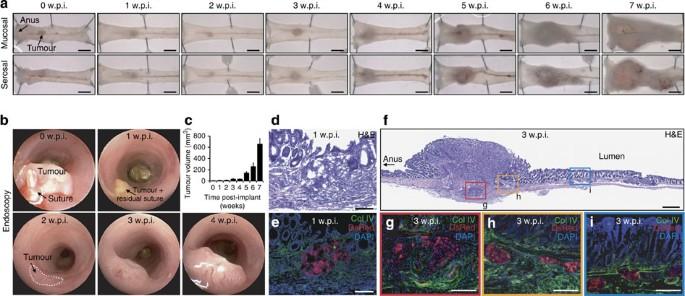Figure 2: Lumen-implanted colorectal tumours incorporate within the mucosa and eventually invade through the colon wall. (a) Time course of gross colorectal tumour development following lumen implantation. Colons from NOD/SCID mice bearing HCT116-DsRed lumen tumours were harvested at weekly intervals from 0 to 7 weeks post implantation (w.p.i.), opened longitudinally and imaged. Top and bottom panels show mucosal and serosal views of the colon, respectively, with the anus positioned to the left of every panel. Scale bars represent 5 mm. (b) Endoscopy images following HCT116-DsRed lumen implantation. Serial images were captured from the same host from 0 to 4 w.p.i. Dotted line at 2 w.p.i. indicates the perimeter of the implanted tumour. (c) Primary tumour volume following lumen implantation. Number of mice per time point: 0 w.p.i. (n=3), 1 w.p.i. (n=3), 2 w.p.i. (n=6), 3 w.p.i. (n=6), 4 w.p.i. (n=11), 5 w.p.i. (n=15), 6 w.p.i. (n=11), 7 w.p.i. (n=18). Data are represented by the mean and s.e.m. (d,e) Histological analyses of a host colon implanted with an HCT116-DsRed donor tumour at 1 w.p.i., showing (d) haematoxylin and eosin (H&E) staining and (e) collagen IV (Col IV; green), DsRed (red) and 4',6-diamidino-2-phenylindole (DAPI; blue) staining. Scale bars represent 200 μm. (f–i) Histological analyses of a host colon implanted with an HCT116-DsRed donor tumour at 3 w.p.i., showing (f) H&E staining and (g–i) Col IV (green), DsRed (red) and DAPI (blue) staining. Red-, yellow- and blue-boxed areas infare shown enlarged ing–i, respectively. Scale bars represent 500 μm (f) and 100 μm (g–i). Figure 2: Lumen-implanted colorectal tumours incorporate within the mucosa and eventually invade through the colon wall. ( a ) Time course of gross colorectal tumour development following lumen implantation. Colons from NOD/SCID mice bearing HCT116-DsRed lumen tumours were harvested at weekly intervals from 0 to 7 weeks post implantation (w.p.i. ), opened longitudinally and imaged. Top and bottom panels show mucosal and serosal views of the colon, respectively, with the anus positioned to the left of every panel. Scale bars represent 5 mm. ( b ) Endoscopy images following HCT116-DsRed lumen implantation. Serial images were captured from the same host from 0 to 4 w.p.i. Dotted line at 2 w.p.i. indicates the perimeter of the implanted tumour. ( c ) Primary tumour volume following lumen implantation. Number of mice per time point: 0 w.p.i. ( n =3), 1 w.p.i. ( n =3), 2 w.p.i. ( n =6), 3 w.p.i. ( n =6), 4 w.p.i. ( n =11), 5 w.p.i. ( n =15), 6 w.p.i. ( n =11), 7 w.p.i. ( n =18). Data are represented by the mean and s.e.m. ( d , e ) Histological analyses of a host colon implanted with an HCT116-DsRed donor tumour at 1 w.p.i., showing ( d ) haematoxylin and eosin (H&E) staining and ( e ) collagen IV (Col IV; green), DsRed (red) and 4',6-diamidino-2-phenylindole (DAPI; blue) staining. Scale bars represent 200 μm. ( f – i ) Histological analyses of a host colon implanted with an HCT116-DsRed donor tumour at 3 w.p.i., showing ( f ) H&E staining and ( g – i ) Col IV (green), DsRed (red) and DAPI (blue) staining. Red-, yellow- and blue-boxed areas in f are shown enlarged in g – i , respectively. Scale bars represent 500 μm ( f ) and 100 μm ( g – i ). Full size image Having developed lumen implantation as a viable technique for generating stage 0 colorectal tumours that progressed to stage II adenocarcinomas, we next assessed tumour-bearing mice for evidence of regional and/or distant metastatic progression corresponding to stage III/IV disease. At 6–7 w.p.i., locoregional spread of tumour cells within the colon wall was prominent, both proximal ( Fig. 3a,f ) and distal ( Fig. 3a–c ) to the primary tumour site ( Fig. 3a,d,e ). Mice also exhibited hematogenous ( Fig. 3g ), lymphatic ( Fig. 3j ) and perineural ( Fig. 3h ) tumour cell invasion. Regional intestinal lymph node metastases were detectable as macroscopic DsRed-positive tumour nodules located adjacent to the serosa, and within the draining lymphatic network that ran parallel to the colon wall ( Figs 3a,i and 4a ). Importantly, mice also presented with macroscopic DsRed-positive metastases in the liver ( Fig. 4b ) and lungs ( Fig. 4c ). To better characterize the timing of macroscopic metastasis manifestation, we performed a temporal assessment of metastatic burden via gross examination and determined that macrometastases primarily presented an ~4 w.p.i. ( Fig. 4d ). However, macrometastasis presentation does not yield information regarding the precise timing of microscopic disease dissemination. Therefore, we dissociated entire livers, lungs and intestinal marginal vascular tracts to single cells and monitored for DsRed-positive tumour cells by flow cytometry. Disseminated tumour cells were primarily detectable at ~3 w.p.i., one week before the manifestation of gross macrometastases ( Fig. 4e ). We confirmed the presence of disseminated tumour cells within the livers and lungs at 3 w.p.i. by DsRed immunofluorescence, despite the absence of detectable disease at either the gross or histopathological level ( Supplementary Fig. 3b,c ). These findings demonstrate lumen implantation of HCT116 colorectal tumours to be a viable in vivo model that metastasizes in a temporal fashion to regional and distant sites relevant to the human disease. 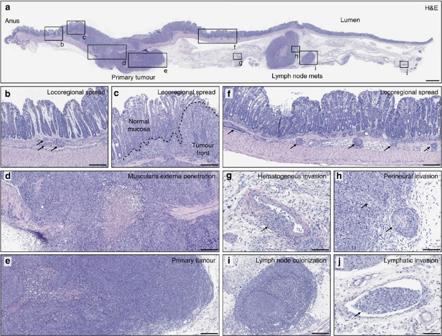Figure 3: Lumen-implanted colorectal tumours exhibit locoregional spread as well as hematogenous and lymphatic vascular invasion. (a–j) Haematoxylin and eosin (H&E) staining of a colon from a NOD/SCID mouse bearing a lumen-implanted HCT116-DsRed tumour at 6 w.p.i. Boxed areas inaare shown enlarged inb–j, demonstrating (b) locoregional spread distal to the primary tumour indicated by arrows, (c) locoregional spread of a tumour migratory front into the normal mucosa outlined by a dotted line, (d) muscularis externa penetration, (e) primary tumour viability, (f) locoregional spread proximal to the primary tumour indicated by arrows, (g) hematogenous invasion indicated by an arrow, (h) perineural invasion indicated by arrows, (i) regional lymph node colonization and (j) lymphatic invasion indicated by an arrow. Scale bars represent 1 mm (a), 200 μm (b–f,i) and 100 μm (g,h,j). Figure 3: Lumen-implanted colorectal tumours exhibit locoregional spread as well as hematogenous and lymphatic vascular invasion. ( a – j ) Haematoxylin and eosin (H&E) staining of a colon from a NOD/SCID mouse bearing a lumen-implanted HCT116-DsRed tumour at 6 w.p.i. Boxed areas in a are shown enlarged in b – j , demonstrating ( b ) locoregional spread distal to the primary tumour indicated by arrows, ( c ) locoregional spread of a tumour migratory front into the normal mucosa outlined by a dotted line, ( d ) muscularis externa penetration, ( e ) primary tumour viability, ( f ) locoregional spread proximal to the primary tumour indicated by arrows, ( g ) hematogenous invasion indicated by an arrow, ( h ) perineural invasion indicated by arrows, ( i ) regional lymph node colonization and ( j ) lymphatic invasion indicated by an arrow. Scale bars represent 1 mm ( a ), 200 μm ( b – f , i ) and 100 μm ( g , h , j ). 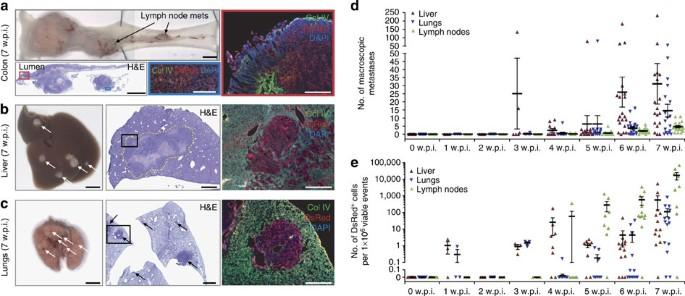Figure 4: Lumen-implanted colorectal tumours generate regional metastases in the intestinal lymph nodes and distant metastases in the liver and lungs. (a–c) Metastasis in a NOD/SCID mouse bearing an HCT116-DsRed lumen tumour at 7 w.p.i. Shown are (a) a gross colon with arrows indicating lymph node metastases, the bottom-left panel showing histological staining by haematoxylin and eosin (H&E), and the blue- and red-boxed areas shown enlarged in the bottom-middle and -right panels, respectively, and stained for Col IV (green), DsRed (red) and 4',6-diamidino-2-phenylindole (DAPI) (blue), (b) liver with arrows indicating metastases, the middle panel showing histological staining by H&E, the dotted line indicating metastatic nodule perimeter, and the boxed area shown enlarged in the right panel and stained for Col IV (green), DsRed (red) and DAPI (blue), (c) lungs with arrows indicating metastases, the middle panel showing histological staining by H&E, arrows indicating metastatic nodules, and the boxed area shown enlarged in the right panel and stained for Col IV (green), DsRed (red) and DAPI (blue). Scale bars represent 4 mm (gross colon, liver, lungs and colon H&E), 1 mm (liver and lung H&E), 400 μm (colon and lung immunostaining) and 200 μm (liver and lymph node immunostaining). (d) Number of macroscopic metastases within the intestinal lymph nodes, liver and lungs following lumen implantation. Number of mice: 0 w.p.i. (n=14), 1 w.p.i. (n=3), 2 w.p.i. (n=6), 3 w.p.i. (n=6), 4 w.p.i. (n=11), 5 w.p.i. (n=15), 6 w.p.i. (n=20), 7 w.p.i. (n=18). (e) DsRed-positive tumour cell burden within the intestinal lymph nodes, liver and lungs following lumen implantation. Data are expressed as the number of DsRed-positive tumour cells per 1 × 106viable events. Number of mice: 0 w.p.i. (n=14), 1 w.p.i. (n=3), 2 w.p.i. (n=3), 3 w.p.i. (n=3), 4 w.p.i. (n=8), 5 w.p.i. (n=8), 6 w.p.i. (n=13), 7 w.p.i. (n=14). Each point indanderepresents data from an individual mouse. Means±s.e.m. are also shown. Full size image Figure 4: Lumen-implanted colorectal tumours generate regional metastases in the intestinal lymph nodes and distant metastases in the liver and lungs. ( a – c ) Metastasis in a NOD/SCID mouse bearing an HCT116-DsRed lumen tumour at 7 w.p.i. Shown are ( a ) a gross colon with arrows indicating lymph node metastases, the bottom-left panel showing histological staining by haematoxylin and eosin (H&E), and the blue- and red-boxed areas shown enlarged in the bottom-middle and -right panels, respectively, and stained for Col IV (green), DsRed (red) and 4',6-diamidino-2-phenylindole (DAPI) (blue), ( b ) liver with arrows indicating metastases, the middle panel showing histological staining by H&E, the dotted line indicating metastatic nodule perimeter, and the boxed area shown enlarged in the right panel and stained for Col IV (green), DsRed (red) and DAPI (blue), ( c ) lungs with arrows indicating metastases, the middle panel showing histological staining by H&E, arrows indicating metastatic nodules, and the boxed area shown enlarged in the right panel and stained for Col IV (green), DsRed (red) and DAPI (blue). Scale bars represent 4 mm (gross colon, liver, lungs and colon H&E), 1 mm (liver and lung H&E), 400 μm (colon and lung immunostaining) and 200 μm (liver and lymph node immunostaining). ( d ) Number of macroscopic metastases within the intestinal lymph nodes, liver and lungs following lumen implantation. Number of mice: 0 w.p.i. ( n =14), 1 w.p.i. ( n =3), 2 w.p.i. ( n =6), 3 w.p.i. ( n =6), 4 w.p.i. ( n =11), 5 w.p.i. ( n =15), 6 w.p.i. ( n =20), 7 w.p.i. ( n =18). ( e ) DsRed-positive tumour cell burden within the intestinal lymph nodes, liver and lungs following lumen implantation. Data are expressed as the number of DsRed-positive tumour cells per 1 × 10 6 viable events. Number of mice: 0 w.p.i. ( n =14), 1 w.p.i. ( n =3), 2 w.p.i. ( n =3), 3 w.p.i. ( n =3), 4 w.p.i. ( n =8), 5 w.p.i. ( n =8), 6 w.p.i. ( n =13), 7 w.p.i. ( n =14). Each point in d and e represents data from an individual mouse. Means±s.e.m. are also shown. Full size image We next determined if the lumen implantation procedure would yield similar progression and metastasis profiles if colorectal tumours of different origin were used as donors. To this end, we used the well-differentiated primary human CRC-derived LS174T cell line. We transduced LS174T cells with a lentivirus encoding DsRed, generated LS174T-DsRed subcutaneous tumours in a donor mouse and transplanted donor tumour fragments onto the mucosal surface of host mouse colons. Similar to lumen-implanted HCT116 tumours, lumen-implanted LS174T tumours initially grew within the mucosal layer and eventually invaded through the colon wall, such that the bulk of the primary tumour burden was situated on the serosal side of the wall at the 8 w.p.i. harvest endpoint ( Supplementary Fig. 4a,b ). Notably, metastatic outgrowths in the liver, lungs and regional lymph nodes were also apparent in this model, albeit with a longer latency than in the HCT116 tumour-bearing mice ( Supplementary Fig. 4a,c–e ). We further validated the utility of this model using primary human patient CRC tumours as donors, demonstrating that lumen-implanted tumours from a stage II patient remained non-metastatic whereas lumen-implanted tumours from a stage III patient gave rise to intestinal lymph node metastases ( Supplementary Fig. 4f–h ). These findings highlight the clinical relevance of disease progression in the lumen implant model, and further raise the possibility that lumen implantation of patient-derived CRC tumours may hold predictive value with respect to eventual metastasis presentation. Selective metastasis of lumen-implanted colorectal tumours In the clinic, certain tumour types specifically metastasize to certain organs [20] . Indeed, CRC predominantly metastasizes to the regional intestinal lymph nodes, liver and lungs, whereas other organs are largely spared [21] . To determine whether the lumen implantation model would accurately recapitulate the preferential target organ specificity observed in humans, we assessed metastatic tumour burden at 6–7 w.p.i. in various internal organs by both macroscopic examination and DsRed-positive tumour cell flow cytometry. NOD/SCID mice bearing lumen-implanted HCT116-DsRed tumours preferentially developed metastases in the liver, lungs and intestinal lymph nodes, with minimal metastatic burden detectable in the adrenal gland, kidney, spleen, brain and bone marrow ( Fig. 5a,b and Supplementary Fig. 5a ). This preferential target organ homing was maintained when HCT116 tumours were implanted into the colons of the more highly immunocompromised NOD/SCID interleukin-2 receptor gamma chain null (NSG) mouse strain ( Fig. 5c–g ), despite a significant increase in metastatic tumour burden within the liver, lungs and intestinal lymph nodes in NSG ( Fig. 5a,b ) compared with NOD/SCID ( Figs 4b,c and 5a,b ) mice. This enhancement of primary tumour metastatic potential can be attributed in part to the lack of natural-killer cell activity in NSG mice, consistent with previous reports [22] , [23] . Importantly, we never observed peritoneal carcinomatosis in any of our transplanted NOD/SCID or NSG host mice—a feature that is widespread in the previously reported CRC models to date [14] , [15] , [16] , [17] . Given that peritoneal carcinomatosis is not a common manifestation in human CRC [18] , our findings further highlight the relevance and advantage of our metastatic CRC model over those that have been reported in the literature. 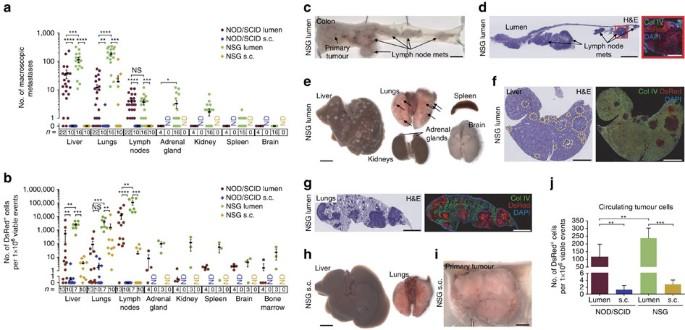Figure 5: Lumen-implanted colorectal tumours form metastases in selective target organs. (a,b) Number of (a) macroscopic metastases or (b) DsRed-positive tumour cells following lumen or subcutaneous (s.c.) implantation of HCT116-DsRed tumours into NOD/SCID or NSG mice. Each point represents data from an individual mouse. Means±s.e.m. are also shown. *P<0.05; **P<0.01; ***P<0.001; ****P<0.0001;t-test. NS, not significant. ND, not determined. (c–g) Metastasis assessment of an NSG mouse bearing an HCT116-DsRed lumen tumour at 7 w.p.i. Shown are (c) a gross colon with arrows indicating the primary tumour and regional lymph node metastases, (d) colon histology with the left panel stained by haematoxylin and eosin (H&E), the boxed area shown enlarged in the right panel and stained for Col IV (green), DsRed (red) and 4',6-diamidino-2-phenylindole (DAPI) (blue), and arrows indicate regional lymph node metastases, (e) various organs from the same host with liver metastases clearly evident and lung metastases indicated by arrows, (f) liver histology with the left panel stained by H&E, the right panel stained for Col IV (green), DsRed (red) and DAPI (blue), and dotted lines indicating the perimeter of liver metastatic nodules, and (g) lung histology with the left panel stained by H&E and the right panel stained for Col IV (green), DsRed (red) and DAPI (blue). (h,i) Metastasis assessment of an NSG mouse bearing an HCT116-DsRed s.c. tumour at 7 w.p.i., showing (h) liver and lungs and (i) the associated primary s.c. tumour. (j) Circulating tumour cell number at 6–7 w.p.i. following lumen or s.c. implantation of HCT116-DsRed tumours into NOD/SCID or NSG mice. Data are represented by the mean and s.e.m., and are expressed as the number of DsRed-positive tumour cells in the blood per 1 × 106viable events. Number of mice: NOD/SCID lumen (n=12); NOD/SCID s.c. (n=9); NSG lumen (n=9); NSG s.c. (n=10). **P<0.01; ***P<0.001;t-test. Scale bars represent 5 mm (c), 4 mm (d,e,h,i), 2 mm (f,g), and 1 mm (d—boxed area). Figure 5: Lumen-implanted colorectal tumours form metastases in selective target organs. ( a , b ) Number of ( a ) macroscopic metastases or ( b ) DsRed-positive tumour cells following lumen or subcutaneous (s.c.) implantation of HCT116-DsRed tumours into NOD/SCID or NSG mice. Each point represents data from an individual mouse. Means±s.e.m. are also shown. * P <0.05; ** P <0.01; *** P <0.001; **** P <0.0001; t -test. NS, not significant. ND, not determined. ( c – g ) Metastasis assessment of an NSG mouse bearing an HCT116-DsRed lumen tumour at 7 w.p.i. Shown are ( c ) a gross colon with arrows indicating the primary tumour and regional lymph node metastases, ( d ) colon histology with the left panel stained by haematoxylin and eosin (H&E), the boxed area shown enlarged in the right panel and stained for Col IV (green), DsRed (red) and 4',6-diamidino-2-phenylindole (DAPI) (blue), and arrows indicate regional lymph node metastases, ( e ) various organs from the same host with liver metastases clearly evident and lung metastases indicated by arrows, ( f ) liver histology with the left panel stained by H&E, the right panel stained for Col IV (green), DsRed (red) and DAPI (blue), and dotted lines indicating the perimeter of liver metastatic nodules, and ( g ) lung histology with the left panel stained by H&E and the right panel stained for Col IV (green), DsRed (red) and DAPI (blue). ( h , i ) Metastasis assessment of an NSG mouse bearing an HCT116-DsRed s.c. tumour at 7 w.p.i., showing ( h ) liver and lungs and ( i ) the associated primary s.c. tumour. ( j ) Circulating tumour cell number at 6–7 w.p.i. following lumen or s.c. implantation of HCT116-DsRed tumours into NOD/SCID or NSG mice. Data are represented by the mean and s.e.m., and are expressed as the number of DsRed-positive tumour cells in the blood per 1 × 10 6 viable events. Number of mice: NOD/SCID lumen ( n =12); NOD/SCID s.c. ( n =9); NSG lumen ( n =9); NSG s.c. ( n =10). ** P <0.01; *** P <0.001; t -test. Scale bars represent 5 mm ( c ), 4 mm ( d , e , h , i ), 2 mm ( f , g ), and 1 mm ( d —boxed area). Full size image To determine if HCT116 cells were capable of metastasis regardless of implantation site, we implanted HCT116-DsRed cells subcutaneously in both NOD/SCID and NSG mice and assessed metastatic burden. Subcutaneously-implanted tumours did not readily metastasize compared with their lumen-implanted counterparts, in both NOD/SCID ( Fig. 5a,b and Supplementary Fig. 5b,c ) and NSG ( Fig. 5a,b,h,i ) mouse strains. Histological assessment of size-matched and time-matched 6 w.p.i. HCT116 tumours in NOD/SCID mice revealed that although subcutaneously-implanted tumours were highly necrotic, lumen-implanted tumours were almost completely devoid of necrosis ( Supplementary Fig. 5d,e ). This lack of necrosis may be attributed to enhanced vascularization in lumen-implanted tumours, as evidenced by MECA-32 immunostaining for endothelial cells ( Supplementary Fig. 5f–h ), which in turn may be attributed to enhanced vascular density at the mucosal versus subcutaneous implantation sites. Given that lumen-implanted tumours exhibited increased vascular density concommitant with increased metastasis relative to subcutaneously-implanted tumours, we sought to determine whether circulating tumour cell number could be reflective of metastatic potential, as has been reported in the clinic [24] . Consistently, lumen-implanted tumours gave rise to ~100-times more circulating tumour cells than subcutaneously-implanted tumours in both NOD/SCID and NSG mice, with lumen-implanted NSG mice exhibiting an ~2.5-fold greater circulating tumour cell number than lumen-implanted NOD/SCID mice ( Fig. 5j ). Hence robust metastasis formation following lumen implantation correlated with increased primary tumour vascularization, which in turn correlated with enhanced tumour cell entry into the circulation. Taken together, these findings do not support an inherent metastatic phenotype in HCT116 tumours, but rather highlight the fact that the same tumour cells can exhibit drastically different metastatic capacity dependent upon their primary tumour microenvironment. Liver metastasis independent of a lymph node intermediary To date, no in vivo model of CRC has demonstrated predictable and reproducible distant metastatic outgrowth within relevant target organs from an orthotopically-established primary colorectal tumour [2] , [3] , [4] , [5] . The lack of available models has precluded investigations into the route(s) of metastatic spread to distant organs. In the clinic, it is unknown whether colorectal metastases in the liver arise secondary to an initial colonization of the regional intestinal lymph nodes, or whether these liver metastases arise via direct hematogenous spread from the primary tumour, independent of lymph node metastatic growth [1] . The first hypothesis is supported by the observations that (i) staging criteria are based on the degree to which the cancer has spread; clinical presentation of intestinal lymph node metastases alone is indicative of stage III disease whereas the presence of liver metastases are cause for the more advanced stage IV diagnosis [25] , (ii) high co-incidence has been reported for distant liver metastases and intestinal lymph node metastases [26] , (iii) primary tumour lymphatic vessel density correlates with metastasis to both the lymph nodes and liver [27] , and (iv) tumour cell entry into the lymphatics is presumably easier than entry into the hematogenous vasculature due to a discontinuous basement membrane and a lack of pericyte coverage [28] . Several observations support the second hypothesis, including (i) that some CRC patients present with liver metastases in the absence of lymph node involvement [26] , (ii) that surgical removal of an increased number of draining intestinal lymph nodes in stage III CRC patients may not improve overall survival [29] , [30] , [31] , and (iii) that venous invasion of the primary tumour is an independent prognostic indicator of distant liver metastasis development in CRC [32] . Having developed lumen implantation as a metastatic CRC model, we were uniquely positioned to interrogate dissemination routes. In patients a correlation exists between the presence/absence of lymph node metastases and the presence/absence of liver metastases [26] ; however, whether the number of involved lymph nodes correlates with the number of liver metastatic nodules remains unknown. In both our NOD/SCID and NSG lumen implant models, lymph node metastatic burden (both total number of involved lymph nodes and total DsRed-positive tumour cell burden within the lymph nodes) did not correlate with liver metastatic burden ( Fig. 6a,b ), suggesting that dissemination to the lymph nodes and liver might occur via distinct routes. 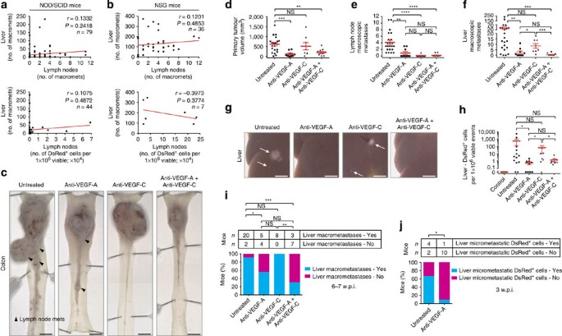Figure 6: Colorectal cancer metastases in the liver can manifest in the absence of an intestinal lymph node metastatic intermediary. (a,b) Correlations between lymph node metastatic burden and liver metastatic burden in mice bearing lumen-implanted HCT116-DsRed tumours. Data are the total number of macroscopic liver metastases versus either the total number of macroscopic lymph node metastases or the total number of DsRed-positive tumour cells within the lymph nodes, in (a) NOD/SCID mice from 1–7 w.p.i. or (b) NSG mice from 5–7 w.p.i. (c–i) Effect of targeting angiogenesis and/or lymphangiogenesis on the formation of regional lymph node metastases and distant liver metastases in NOD/SCID mice bearing lumen-implanted HCT116-DsRed tumours at 6–7 w.p.i. Shown are (c) gross serosal images of colons with arrowheads indicating intestinal lymph node metastases, (d) primary tumour volumes, (e) number of lymph node macroscopic metastases, (f) number of liver macroscopic metastases, (g) gross images of livers with arrows indicating metastases, (h) DsRed-positive tumour cell burden within the liver alongside control analyses from non-tumour-bearing mice (n=8), with data expressed as the number of DsRed-positive tumour cells per 1 × 106viable events and (i) contingency analyses comparing the number of mice with or without liver macrometastases at 6–7 w.p.i., with data expressed as the percentage of mice in each category. Number of mice per treatment condition: untreated (n=22 ford–f, andn=13 forhandi), anti-VEGF-A (n=9), anti-VEGF-C (n=8), anti-VEGF-A/C (n=10 ford–f, andn=9 forhandi). (j) Contingency analysis comparing the number of mice with or without liver micrometastatic DsRed-positive cells at 3 w.p.i., before macroscopic metastasis manifestation, with data expressed as the percentage of mice in each category. Each point ina,b,d–fandhrepresents data from an individual mouse. Means±s.e.m. are also shown. *P<0.05; **P<0.01; ***P<0.001; ****P<0.0001; group differences—t-test; contingency analyses—Fisher’s exact test. NS, not significant. Scale bars represent 5 mm (c) and 2 mm (g). Figure 6: Colorectal cancer metastases in the liver can manifest in the absence of an intestinal lymph node metastatic intermediary. ( a , b ) Correlations between lymph node metastatic burden and liver metastatic burden in mice bearing lumen-implanted HCT116-DsRed tumours. Data are the total number of macroscopic liver metastases versus either the total number of macroscopic lymph node metastases or the total number of DsRed-positive tumour cells within the lymph nodes, in ( a ) NOD/SCID mice from 1–7 w.p.i. or ( b ) NSG mice from 5–7 w.p.i. ( c – i ) Effect of targeting angiogenesis and/or lymphangiogenesis on the formation of regional lymph node metastases and distant liver metastases in NOD/SCID mice bearing lumen-implanted HCT116-DsRed tumours at 6–7 w.p.i. Shown are ( c ) gross serosal images of colons with arrowheads indicating intestinal lymph node metastases, ( d ) primary tumour volumes, ( e ) number of lymph node macroscopic metastases, ( f ) number of liver macroscopic metastases, ( g ) gross images of livers with arrows indicating metastases, ( h ) DsRed-positive tumour cell burden within the liver alongside control analyses from non-tumour-bearing mice ( n =8), with data expressed as the number of DsRed-positive tumour cells per 1 × 10 6 viable events and ( i ) contingency analyses comparing the number of mice with or without liver macrometastases at 6–7 w.p.i., with data expressed as the percentage of mice in each category. Number of mice per treatment condition: untreated ( n =22 for d – f , and n =13 for h and i ), anti-VEGF-A ( n =9), anti-VEGF-C ( n =8), anti-VEGF-A/C ( n =10 for d – f , and n =9 for h and i ). ( j ) Contingency analysis comparing the number of mice with or without liver micrometastatic DsRed-positive cells at 3 w.p.i., before macroscopic metastasis manifestation, with data expressed as the percentage of mice in each category. Each point in a , b , d – f and h represents data from an individual mouse. Means±s.e.m. are also shown. * P <0.05; ** P <0.01; *** P <0.001; **** P <0.0001; group differences— t -test; contingency analyses—Fisher’s exact test. NS, not significant. Scale bars represent 5 mm ( c ) and 2 mm ( g ). Full size image Given that vascular endothelial growth factors (VEGFs) have critical roles in primary tumour vascularization [33] , with VEGF-A and VEGF-C primarily functioning to promote hematogenous and lymphatic vascularization, respectively [34] , [35] , we assessed the effects of function-blocking antibodies against these factors on metastatic dissemination in our model. To this end, host mice were treated with an anti-VEGF-A antibody [36] or a newly characterized anti-VEGF-C antibody [37] once per week beginning one day before HCT116-DsRed lumen tumour implantation, and metastasis formation was assessed at 6–7 w.p.i. Anti-VEGF-A inhibited macroscopic metastasis formation in the liver ( Fig. 6f,g ), which was confirmed by reductions in both DsRed-positive tumour cell burden ( Fig. 6h ) and the percentage of mice that presented with liver involvement ( Fig. 6i ). Anti-VEGF-A also attenuated ( Fig. 6e ) but did not eliminate ( Fig. 6c ) the growth of gross lymph node metastases, consistent with its role in supporting the growth of metastatic lymph node tumours by promoting angiogenesis [38] . In contrast, despite a near complete abrogation of lymph node metastases ( Fig. 6e ), anti-VEGF-C did not significantly inhibit liver metastasis formation ( Fig. 6f,g ) and accordingly did not reduce DsRed-positive tumour cell burden within the liver ( Fig. 6h ). Anti-VEGF-C also had no effect on the percentage of mice that presented with liver macrometastases ( Fig. 6i ). Combination treatment with anti-VEGF-A and anti-VEGF-C antibodies inhibited both lymph node and liver metastasis formation ( Fig. 6e–g ). We obtained similar results using an alternate LS174T-DsRed lumen implant model ( Supplementary Fig. 6a,b ). To account for differences in primary tumour volume following antibody treatment ( Fig. 6c,d ), we normalized liver metastatic burden to primary tumour volume in all treatment arms and confirmed that anti-VEGF-C-mediated blockade of lymph node metastasis had no impact on liver metastasis formation ( Supplementary Fig. 6c,d ). Although our data support a role for VEGF-A but not VEGF-C in CRC liver metastasis formation, whether anti-VEGF-A inhibited the outgrowth of tumour cells that had already seeded the liver or whether anti-VEGF-A directly inhibited primary tumour cell dissemination to the liver remained uncertain. Indeed, targeting VEGF-A has been well documented to inhibit the outgrowth of CRC cells that had colonized the liver following direct intrasplenic injection [39] . To answer this question, we treated HCT116-DsRed tumour-bearing mice with anti-VEGF-A and assessed livers at 3 w.p.i.—before the manifestation of macroscopic liver metastases ( Fig. 4d,e )—for micrometastatic DsRed-positive tumour cells by flow cytometry. Anti-VEGF-A significantly reduced the number of mice with detectable disseminated tumour cells within the liver ( Fig. 6j ). Taken together, these findings demonstrate that CRC cell metastasis from the primary tumour to the liver can occur via direct hematogenous spread, independent of a lymph node metastatic intermediary. Despite the availability of numerous mouse CRC models that recapitulate primary disease development, no such model has been suitable for investigating metastatic dissemination routes as the formation of metastatic lesions in these models is rare or nonexistent. We have developed a mouse model of metastatic CRC that gives rise to selective and reliable metastatic outgrowth in applicable target organs. Development of this model allowed us to directly interrogate routes of metastatic spread, and to demonstrate that CRC dissemination to the liver can occur independently of prior lymph node colonization—an issue that has been controversial and until now undemonstrable. These results may have important implications for CRC disease staging, as lymph node-positive stage III disease and distant metastasis-positive stage IV disease may be viewed as parallel (rather than sequential) progressions from localized stage II disease. In addition to revealing routes of CRC cell dissemination from the primary tumour to distant sites, our model has the potential to enable the study and targeting of established metastatic lesions in an experimental setting. Indeed, the lack of available mouse metastatic CRC models has proven a barrier to the investigation of metastatic disease drivers and the therapeutic response of lesions that have spontaneously metastasized from a primary tumour. It is becoming increasingly clear that primary CRCs and their subsequent matched liver metastases are both genetically and biologically distinct [40] , [41] , [42] , [43] . As CRC patient mortality is primarily the result of distant metastatic outgrowth, a mandate exists for the interrogation of therapeutic targets present in established metastases—not just the primary tumour. The development of mouse models that accurately reflect the metastatic disease setting is essential to the fulfillment of such a mandate. Our findings represent a significant biological advance in the understanding of CRC disease mechanisms with the potential to foster the discovery of novel therapeutic strategies and interventions. Mice Wild-type C57BL/6J and NOD/SCID female mice (8–12 weeks old) were purchased from Charles River Laboratories. Wild-type NSG female mice (8–12 weeks old; stock number 005557), Apc Min/+ mice (stock number 002020), and 12.4KbVilCre mice (stock number 004586; referred to as Villin-Cre ) were purchased from the Jackson Laboratory. Kras LSLG12D/+ mice were licensed from Tyler Jacks from the Massachusetts Institute of Technology. Apc/Kras compound mutant mice from colony number 4028 were bred with CAG-mRFP1 mice (stock number 005884) purchased from the Jackson Laboratory. Apc/Kras compound mutant mice from colony number 4700 were bred with Rosa26-CAG-LSL-tdTomato mice (stock number 007909) purchased from the Jackson Laboratory. All experiments were approved by the Animal Research Ethics and Protocol Review Committee of Genentech. Cell culture and gene transfer HCT116 and LS174T human CRC-derived cell lines were purchased from ATCC and maintained in complete Roswell Park Memorial Institute (RPMI) medium (RPMI 1640 supplemented with 10% fetal bovine serum, 2 mM glutamine, 100 U ml −1 penicillin and 100 mg ml −1 streptomycin) at 37 °C and 5% CO 2 . Cells were transduced with a TZV-CMV-Discosoma red fluorescent protein (DsRed) lentiviral vector (Open Biosystems) at a multiplicity-of-infection of 10 in complete RPMI medium supplemented with 8 mg ml −1 polybrene for 6 h at 37 °C and 5% CO 2 . After four passages in culture, DsRed-positive cells were isolated by fluorescence-activated cell sorting on a FACSAria (BD Biosciences). Sorted DsRed-positive cells were expanded for 2–3 passages, and then stored in liquid nitrogen. Early passage cells were used for all in vivo experiments. Subcutaneous tumour generation Cell lines were harvested via trypsinization, counted with trypan blue to assess viability, and resuspended in cold complete RPMI medium at a concentration of 100 × 10 6 cells ml −1 . Cold Matrigel (BD Biosciences) was added to the cell suspension at a 1:1 ratio to achieve a final cell concentration of 50 × 10 6 cells ml −1 . NOD/SCID mice were injected with 5 × 10 6 cells in a volume of 100 μl subcutaneously in the left flank. Tumour dimensions were measured using calipers and tumour volume was calculated as 0.523 × length × width × width. For subcutaneous tumours used as donors for the lumen implantation technique, tumours were harvested between 1,000–2,000 mm 3 , necrotic tissue grossly dissected away under a microscope, and the remaining viable tissue divided into 10 mm 3 fragments and placed on ice in complete RPMI medium. Lumen implantation technique Mice were anaesthetized by isoflurane inhalation, placed in a supine position, and the extremities secured to a gauze-covered platform with tape. A blunt-ended hemostat (Micro-Mosquito, No. 13010-12, Fine Science Tools) was inserted ~1 cm into the anus, and the hemostat angled towards the mucosa and opened slightly such that a single mucosal fold could be clasped by closing the hemostat to the first notch. The hemostat was retracted from the anus, and the clasped exteriorized mucosa cleansed with povidone/iodine, rinsed with lactated ringers solution and blotted dry. A donor tumour fragment or intact polyp of ~10 mm 3 was sutured onto the mucosa using absorbable 4-0 Vicryl sutures (Ethicon), ensuring that the suture only penetrated the superficial mucosal layer. After rehydrating the mucosa with phosphate-buffered saline (PBS), the hemostat was released and a blunt gavage needle used to re-insert the exteriorized colon together with the sutured tumour, thus reversing the rectal prolapse. The average tumour implantation distance was 11.8±0.5 mm away from the anus ( n =18). Mortality post surgery was less than 1%, with morbidity at 2–4 w.p.i. attributable to reversible rectal prolapse in less than 5% of mice and morbidity at 7 w.p.i. attributable to weight loss due to increased tumour burden. Tumour take rates for the various donor tumour types and host mouse strains are summarized in Supplementary Table 1 . To minimize tumour dislodgement during defecation, mice were housed on cage floor inserts and fed a 100% rodent liquid diet (AIN-76A, Casein Hydrolysate without fibre; BioServe) from 3 days pre-surgery until 7 days post surgery. Endoscopy Before endoscopic imaging, mice were anesthetized by isoflurane inhalation, placed in a supine position, and their colons evacuated of stool using a gavage needle. Endoscopic imaging equipment consisted of a Hopkins II 0° straight forward 1.9 mm outer diameter telescope encompassed by an examination and protection sheath, an Image-1 high definition three-chip digital camera attached to a Mikata Point Setter telescope holding system, a fibre optic light guide cable connected to a D Light System xenon light source, an electronic CO 2 insufflator to maintain colon insufflation during imaging, and an AIDA Connect high definition documentation system connected to a high definition colour monitor (Karl Storz). Endoscopic videos were reviewed using VLC Media Player (VideoLAN Team) and still images were captured from these videos. Whole organ imaging and macrometastasis evaluation Colons were harvested intact, flushed with PBS, opened longitudinally, pinned down on thin cardboard pieces, and imaged both mucosally and serosally. Livers and lungs were harvested, washed in PBS and imaged. All organs were imaged using a DFC295 colour digital camera (Leica) attached to an M80 stereomicroscope (Leica). Macroscopic metastasis formation was assessed visually using a S4 stereomicroscope (Leica). For the intestinal lymph nodes, the entire intestinal tract from the anus to the stomach was examined for evidence of lymph node involvement, and the number of macrometastases quantified. For the liver and lungs, the entire external surface of whole organs was examined and the number of macrometastases quantified. Following macrometastasis quantification, organs were fixed in 4% paraformaldehyde in PBS overnight. Before overnight fixation in 4% paraformaldehyde, lungs were perfused with 4% paraformaldehyde in PBS. Primary colorectal tumour dimensions were determined using a reference measurement scale and tumour volume was calculated as 0.523 × length × width × width. Tissue digestion and flow cytometry Entire tissues were processed on a GentleMACS dissociator (Miltenyi Biotec), digested in complete RPMI medium supplemented with 1 mg ml −1 collagenase/dispase for 30 min at 37 °C with agitation at 210 r.p.m., and filtered through a 70 μm strainer. Following red blood cell lysis and centrifugation, cells were resuspended in PBS supplemented with 2% fetal bovine serum, 20 mM HEPES and 5 μg ml −1 propidium iodide, filtered into fluorescence-activated cell sorting (FACS) tubes and analysed on a FACSAria flow cytometer (BD Biosystems). For FACS controls, normal tissues from non-tumour-bearing mice were used, and DsRed-positive analysis gates were established such that zero DsRed-positive events were detectable in control tissue specimens. An average of 5 × 10 6 viable events were analysed per specimen. Data were analysed with FlowJo software and expressed as the number of DsRed-positive cells per 1 × 10 6 viable events. Circulating tumour cells Mice were killed by CO 2 inhalation. Immediately after breathing subsided, the rib cage was splayed open to expose the heart. A syringe fitted with a 27-gauge needle was inserted into the right chamber of the heart, and ~500 μl of blood was withdrawn. Blood was immediately transferred to EDTA-coated Microtainer tubes (BD Biosciences). Following red blood cell lysis, blood samples were resuspended in PBS supplemented with 2% fetal bovine serum, 20 mM HEPES, and 5 μg ml −1 propidium iodide and analysed by flow cytometry. For FACS controls, blood from non-tumour-bearing mice was used, and DsRed-positive analysis gates were established such that zero DsRed-positive events were detectable in control blood specimens. An average of 5 × 10 6 viable events were analysed per specimen. Data were analysed with FlowJo software and expressed as the number of DsRed-positive cells per 1 × 10 6 viable events. Human CRC clinical specimens Freshly resected human colorectal cancer specimens were obtained from Bio-options Inc., from consenting patients in accordance with federal and state guidelines. Specimens were shipped overnight at 4 °C in Dulbecco’s modified Eagle’s medium containing high glucose supplemented with 10% fetal bovine serum, glutamine, vancomycin, metronidazole, cefotaxime, amphotericin B, penicillin, streptomycin and protease inhibitor cocktail. Specimens were cut into ~10 mm 3 tumour fragments, and individual fragments implanted under the kidney capsule of athymic nu/nu male mice (6–8 weeks old) purchased from Harlan Sprague Dawley. Six months post implantation, tumours that grew under the kidney capsule were re-implanted subcutaneously to generate a subcutaneous donor tumour source. Donor tumour fragments of ~10 mm 3 were implanted into the colonic lumens of NOD/SCID or NSG mice. Anti-VEGF-A and anti-VEGF-C antibodies Mice were dosed in vivo with anti-VEGF-A clone G6-31 monoclonal antibody [36] and/or anti-VEGF-C clone VC4.5 monoclonal antibody [37] . VC4.5 was isolated from synthetic phage antibody libraries built on a single framework [44] by selection against a matured form of human VEGF-C (R&D Systems). One positive clone VC4 as full-length IgG was verified to block the interaction between human VEGF-C and human VEGFR3, inhibit VEGF-C-induced cell activity and cross-bind murine VEGF-C. VC4 was further affinity-improved to VC4.5 with phage display selection [45] and shown to improve the potency of blocking VEGF-C from receptor binding and cell signalling. VC4.5 exhibits similar affinity towards human and murine VEGF-C (Kd=0.3–1 nM) as determined by surface plasmon resonance measurement using BIAcore instruments by immobilizing either VC4.5 IgG or VEGF-C on the chip. Vascular targeting One day before lumen implantation, NOD/SCID mice were treated with the function-blocking monoclonal antibodies anti-VEGF-A (G6-31; 5 mg kg −1 in PBS) and/or anti-VEGF-C (VC4.5; 40 mg kg −1 in PBS) by intraperitoneal injection. On day 0, HCT116-DsRed or LS174T-DsRed tumour fragments were implanted onto the colonic mucosa. Antibodies were administered once per week. Histopathology and immunostaining Tissues were fixed in 4% paraformaldehyde in PBS overnight, rinsed in PBS, cryoprotected in 30% sucrose in PBS overnight at 4 °C, embedded in optimal cutting temperature compound and frozen at −80 °C, and sectioned at 8 μm. For histopathological analyses, tissue sections were stained with haematoxylin and eosin using a Jung Autostainer XL (Leica), and whole tissue section scans were acquired using a NanoZoomer (Hamamatsu). For immunohistochemical analyses, tissue sections were incubated with primary antibody overnight at 4 °C and secondary antibody for 30 min at room temperature. Primary antibodies used were rabbit anti-collagen IV (polyclonal ab6586; Abcam; 1:100 dilution), goat anti-DsRed (polyclonal sc-33354; Santa Cruz Biotechnology; 1:100 dilution) and rat anti-pan endothelial cell marker (clone MECA-32; Pharmingen; 2 μg ml −1 ). Secondary antibodies used were conjugated to Alexa Fluor 488 or 594 (Invitrogen). Images were acquired on an Axioplan 2 imaging microscope (Zeiss) with an ORCA-ER digital camera (Hamamatsu). Vascular density was expressed as a ratio of the MECA-32-positive vascular area over the total 4',6-diamidino-2-phenylindole-positive viable tumour area multiplied by 100. Histology specimens were reviewed by a trained pathologist with CRC disease expertise. Statistical analyses Group differences were evaluated by two-tailed Student’s t -test. Correlations were evaluated by Pearson correlation coefficients. Contingency analyses were evaluated by two-sided Fisher’s exact test, using actual mouse numbers as input data. For Kaplan–Meier survival analyses, P -values were computed using the Log-rank test, and hazard ratios were computed using Apc Min/+ ; Villin-Cre mice as the comparator. P -values less than 0.05 were considered significant. How to cite this article: Enquist, I. B. et al. Lymph node-independent liver metastasis in a model of metastatic colorectal cancer. Nat. Commun. 5:3530 doi: 10.1038/ncomms4530 (2014).